Cancer-associated fibroblasts regulate the plasticity of lung cancer stemness via paracrine signalling Cancer stem cells (CSCs) are a promising target for treating cancer, yet how CSC plasticity is maintained in vivo is unclear and is difficult to study in vitro . Here we establish a sustainable primary culture of Oct3/4(+)/Nanog(+) lung CSCs fed with CD90(+) cancer-associated fibroblasts (CAFs) to further advance our knowledge of preserving stem cells in the tumour microenvironment. Using transcriptomics we identify the paracrine network by which CAFs enrich CSCs through de-differentiation and reacquisition of stem cell-like properties. Specifically, we find that IGF1R signalling activation in cancer cells in the presence of CAFs expressing IGF-II can induce Nanog expression and promote stemness. Moreover, this paracrine signalling predicts overall and relapse-free survival in stage I non-small cell lung cancer (NSCLC) patients. IGF-II/IGF1R signalling blockade inhibits Nanog expression and attenuates cancer stem cell features. Our data demonstrate that CAFs constitute a supporting niche for cancer stemness, and targeting this paracrine signalling may present a new therapeutic strategy for NSCLC. Lung cancer is the most common fatal malignancy worldwide [1] . Owing to the success of driver gene identification and specific targeted therapy, many lung cancer patients show good initial responses. However, most patients eventually develop drug resistance and relapse within 1 year [2] , [3] . Current anticancer strategies indicate that most traditional interventions are aimed at cancer cells of an unspecified type, although solid tumours represent an organized, heterogenous cell population [4] . The complicated cell–cell interactions that form the tumour microenvironment (or niche) involve a small population of cells termed cancer stem/initiating cells (cancer stem cells; CSCs). These cells are believed to represent the cause of most malignant tumours, and both CSCs and the tumour niche play major roles in cancer recurrence, metastasis and drug resistance [5] , [6] , [7] , [8] . Thus, specifically targeting the tumour microenvironment or CSCs has recently been suggested as a new strategy for anticancer therapy [9] , [10] , [11] , [12] . The CSC theory is based on the presence of a sub-population of tumorigenic stem-like cells with true multipotency and asymmetric division ability, which enable these cells to self-renew, differentiate into specialized cell types and develop into cancer [7] , [13] . The phenotype of ‘cancer stemness’ may be the driving force behind carcinogenesis [5] , and CSCs may contribute to chemo- or radioresistance and metastasis [11] , [14] , [15] . Increasing evidence shows that CSCs are not only present in leukaemia but also in various solid tumours, including lung cancer [12] , [16] , [17] . Although lung CSCs can be isolated from side populations (SPs) through specific markers such as CD133 and aldehyde dehydrogenase (ALDH) [18] , [19] , [20] , it remains difficult to maintain the stemness characteristics of CSCs in vitro for detailed studies [18] , [21] . To maintain a quiescent state, most stem cells (for example, embryonic, induced pluripotent stem cells and even lung stem cells) depend on direct contact in the microenvironment or the presence of ‘feeder cells’ [22] , [23] , [24] , [25] , [26] , [27] . Interestingly, recent discoveries have also indicated that the tumour microenvironment may promote and enhance tumorigenicity under inflammatory or transforming growth factor-beta (TGF-β) signals [28] , [29] , [30] . In human lung cancer, the tumour microenvironment contains an abundance of cancer-associated fibroblasts (CAFs) [31] . CAFs differ morphologically and functionally from normal fibroblasts (NFs), and they are activated and responsive to crosstalk with cancer cells during carcinogenesis [32] , [33] . Such interactions may create a niche for tumour growth and metastasis [6] , [11] , [34] , [35] , [36] , [37] , [38] , and recent studies have shown that CAFs may stimulate epithelial–mesenchymal transition (EMT)-driven cancer stemness in prostate cancer [39] , [40] through reciprocal activation between CAF and cancer cells [39] . However, it remains unclear whether CAFs contribute to stemness maintenance or cell plasticity [40] , [41] . In this study, CAF feeders from clinical lung cancer patients demonstrated a powerful ability to maintain and enrich the CSC population as a sustainable sphere-forming primary lung CSC culture. This CSC/CAF co-culture system should also be useful for subsequent investigations into how the tumour microenvironment maintains cancer stemness, the signalling involved in cancer cell differentiation and even anti-CSC drug development. Most importantly, our findings revealed that CSC growth was regulated in a paracrine manner by CAFs through the insulin-like growth factor-II (IGF-II)/IGF1 receptor (IGF1R)/Nanog pathway; in particular, the inhibition of IGF1R signalling using a specific antibody or inhibitors could suppress cancer stemness and tumour growth. Finally, we confirmed these results in a cohort of 80 stage I non-small cell lung cancer (NSCLC) patients and determined the pathophysiological significance of IGF-II/IGF1R/Nanog paracrine signalling on lung cancer progression. Together, these findings suggest that tumour microenvironment CAFs may play an important role in maintaining cancer stemness. 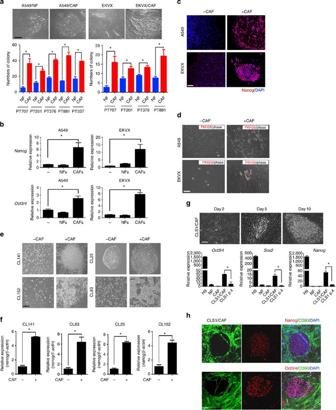Figure 1: The role of CAFs or NFs as feeders to promote tumorigenicity and upregulate stemness markers in lung cancer cells. (a) The colony-formation ability of A549 and EKVX cell lines co-cultured with paired CAFs or NFs from different lung cancer patients (N=4~5 patients, PT707, 201, 376, 881 and 337). Scale bar, 100 μm. (b) RT Q–PCR analysis of the stem cell markers Oct3/4 and Nanog in A549 and EKVX cells cultured with or without NFs and CAFs (N=3~4 patients, PT707, 201, 376 and 881). (c) Immunofluorescent staining for Nanog in A549 and EKVX cells cultured with or without CAFs. The nuclei were stained with DAPI. Scale bar, 100 μm. (d) PKH26 retention assay with A549 and EKVX cells. The cells were pre-stained with the PKH26 red fluorescent dye, and the cells were cultured with or without CAFs. Scale bar, 100 μm. (e) Primary cultured lung cancer cell lines (CL141, CL83, CL25 and CL152) were co-cultured with CAFs, and the cancer cell lines that formed spheroid-like colonies were examined. Scale bar, 200 μm.(f) RT Q–PCR analysis of the stem cell marker Nanog in CL141, CL83, CL25 and CL152 cells cultured with or without CAFs (N=3). (g) Lung CSCs (CLS1) derived from lung cancer tissue formed spheres after culturing with CAFs for 2–10 days (upper panel). RT Q–PCR analysis of Oct3/4, Sox2 and Nanog expression in CLS1 cells. RNA was extracted from the CLS1 spheres cultured with CAFs (CLS1/CAF co-culture) or CLS1 cells cultured without CAFs after passage 4 (CLS1 p4). An embryonic stem cell line, H9, was used as the positive control, and CAFs or NFs were used as the feeder cell controls (lower panel;N=3). (h) Immunofluorescence characterization of CLS1 cells and CAFs; the CLS1 cells expressed Oct3/4 and Nanog, whereas CAFs expressed CD90. The nuclei were stained with DAPI. Scale bar, 100 μm. The data represent the mean±s.d. and were tested for significance using (a) two-way analysis of variance with Tukey’spost hoccorrections or (b–g) the Student’st-test; *P<0.05. The data are representative of at least three independent biological experiments, with three or more replicates in each experiment. CAFs from primary lung tumours support lung CSC growth To investigate whether CAFs from NSCLC patients ( Supplementary Table 1 ) could provide the niche for cancer stemness, we cultured CAFs from tumour tissues as feeders to examine stemness characteristics in A549 and EKVX lung cell lines and primary lung cancer cells (CL25, CL83, CL141 and CL152; Fig. 1 ). We demonstrated that CAFs outperformed the paired NFs in terms of their ability to promote sphere-forming activity ( Fig. 1a ). Moreover, these spheres were isolated through laser-capture ( Supplementary Fig. 1 ) and showed higher expression levels of the stemness markers Oct3/4 and Nanog when co-cultured with CAFs but not NFs ( Fig. 1b ). The CAF-co-cultured cancer cells also showed higher immunostaining for the stemness marker Nanog ( Fig. 1c ). Importantly, these stemness markers have been reported to correlate with carcinogenesis and poor clinical outcome [42] , [43] . PKH26-retaining cells were only observed in cancer cells co-cultured with CAFs ( Fig. 1d ), and Fig. 1e and f show that the sphere-forming ability and expression of Nanog in cancer cells enhanced by CAFs were not only observed in cancer cell lines but also in primary lung cancer cells (CL25, CL83, CL141 and CL152) derived from lung adenocarcinoma patients. Figure 1: The role of CAFs or NFs as feeders to promote tumorigenicity and upregulate stemness markers in lung cancer cells. ( a ) The colony-formation ability of A549 and EKVX cell lines co-cultured with paired CAFs or NFs from different lung cancer patients ( N =4~5 patients, PT707, 201, 376, 881 and 337). Scale bar, 100 μm. ( b ) RT Q–PCR analysis of the stem cell markers Oct3/4 and Nanog in A549 and EKVX cells cultured with or without NFs and CAFs ( N =3~4 patients, PT707, 201, 376 and 881). ( c ) Immunofluorescent staining for Nanog in A549 and EKVX cells cultured with or without CAFs. The nuclei were stained with DAPI. Scale bar, 100 μm. ( d ) PKH26 retention assay with A549 and EKVX cells. The cells were pre-stained with the PKH26 red fluorescent dye, and the cells were cultured with or without CAFs. Scale bar, 100 μm. ( e ) Primary cultured lung cancer cell lines (CL141, CL83, CL25 and CL152) were co-cultured with CAFs, and the cancer cell lines that formed spheroid-like colonies were examined. Scale bar, 200 μm. ( f ) RT Q–PCR analysis of the stem cell marker Nanog in CL141, CL83, CL25 and CL152 cells cultured with or without CAFs ( N =3). ( g ) Lung CSCs (CLS1) derived from lung cancer tissue formed spheres after culturing with CAFs for 2–10 days (upper panel). RT Q–PCR analysis of Oct3/4, Sox2 and Nanog expression in CLS1 cells. RNA was extracted from the CLS1 spheres cultured with CAFs (CLS1/CAF co-culture) or CLS1 cells cultured without CAFs after passage 4 (CLS1 p4). An embryonic stem cell line, H9, was used as the positive control, and CAFs or NFs were used as the feeder cell controls (lower panel; N =3). ( h ) Immunofluorescence characterization of CLS1 cells and CAFs; the CLS1 cells expressed Oct3/4 and Nanog, whereas CAFs expressed CD90. The nuclei were stained with DAPI. Scale bar, 100 μm. The data represent the mean±s.d. and were tested for significance using ( a ) two-way analysis of variance with Tukey’s post hoc corrections or ( b – g ) the Student’s t -test; * P <0.05. The data are representative of at least three independent biological experiments, with three or more replicates in each experiment. Full size image Lung CSC cell line established using CAFs as feeder cells Conventional in vitro techniques used for cancer cell isolation have limitations because they cannot enrich and maintain CSCs. To overcome these limitations, we attempted to use CAFs isolated from a lung tumour tissue as feeder cells to support CSCs in vitro . These primary lung cancer cells formed spheres when co-cultured with CAFs ( Supplementary Fig. 2a ), and a sphere-forming lung CSC line, CLS1, was established. As shown in Fig. 1g , a single CLS1 cell formed a sphere within 10 days of subculturing with CAFs, showing high expression levels of Nanog, Sox2 and Oct3/4 ( Fig. 1g,h ), and demonstrated aneuploidy ( Supplementary Fig. 2b ). In contrast, CAFs displaying a normal karyotype were identified as CD90 positive ( Fig. 1h and Supplementary Fig. 2c ) and expressed the myofibroblast markers α-smooth muscle actin and human leukocyte antigen (HLA)-a, b and c ( Supplementary Fig. 2c ). The CLS1 cells were cloned by limited dilution and subcultured with CAF feeders for further study. Using CAFs as feeder cells, the CLS1 cells were subcultured and maintained their sphere-forming ability with high expression levels of Nanog and Oct3/4 ( Supplementary Fig. 3a ), indicating characteristics of cancer cell stemness. To further assess the cancer stemness of CLS1 cells in vivo , a limited dilution of cancer cells was injected into immunodeficient mice [44] . These results showed that as few as 100 CLS1 cells co-cultured with CAFs could generate xenograft tumours in non-obese diabetic/severe combined immunodeficiency mice, and such tumour-initiating ability was maintained after several passages with CAF feeders ( Supplementary Fig. 3b ). Removal of CAFs from the co-culture reduces stemness CAF-co-cultured CLS1 cells (CLS1/CAF) maintained their cancer stemness phenotype; however, when CAFs were removed during passaging, such cancer stemness characteristics were lost, followed by the downregulation of Oct3/4 and Nanog ( Fig. 2a,b ) as well as a reduction in Oct3/4-positive cells and PKH26-retaining cells ( Fig. 2c ). Most importantly, our data showed that the tumour-initiating frequency of CLS1/CAF was 1/910, and these cells demonstrated highly metastatic activity (12/15), whereas the tumour-initiating capacity and metastatic ability of CLS1 cells was decreased (1/4,137) after 12 passages without CAFs ( Fig. 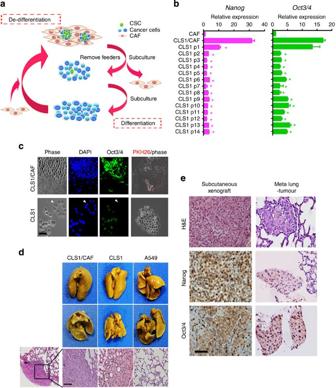Figure 2: Lung CSCs maintain cancer stemness and high tumorigenicity when co-cultured with CAF feeders. (a) Our working hypothesis was that differentiated cancer cells would lose their cancer stemness after CAF removal. (b) RT Q–PCR analysis confirmed that the stemness markersNanogandOct3/4were significantly reduced in CLS1 cells following passages without CAFs (from P1 to P14). The data represent the mean±s.d. (N=3), and the different passages of CLS1 cells with CLS1/CAFs were tested by one-way analysis of variance with Tukey’spost hoccorrections. The data are representative of three independent biological experiments. (c) Immunofluorescence of Oct3/4 in CLS1 cells cultured with (CLS1/CAF) or without CAFs (CLS1) for 5 days. The arrow head shows glandular-type CLS1 cells that lost Oct3/4 staining after CAF removal. The nuclei were stained with DAPI. Retention assay of PKH26 positively stained cells among CLS1 cells. The cells were pre-stained with the PKH26 red fluorescent dye, and the cells were then co-cultured with or without CAFs for 1 week. Arrows mark the CLS1 cells that retained PKH26 fluorescence. Scale bar, 50 μm.(d) Spontaneous lung metastatic nodules of CLS1/CAF (N=15 mice) and CLS1 (N=10 mice) xenograft tumours (upper) were stained with haematoxylin and eosin (H&E; bottom). Scale bar, 100 μm.(e) IHC analysis for Oct3/4 and Nanog expression in a xenograft tumour (subcutaneous and spontaneous lung metastasis tumour) derived from injection of a CLS1 sphere co-cultured with CAFs. Scale bar, 50 μm. 2d , Table 1 and Supplementary Table 2 ). The xenograft tumours showed strong Oct3/4 and Nanog staining in cells at subcutaneous and metastatic sites ( Fig. 2e ). Moreover, these subcutaneous and metastatic lung tumours could be re-cultured, and the primary cultured lung cancer cells from metastatic sites showed a tumorous, spherical phenotype similar to the original CLS1 cells ( Supplementary Fig. 4a ). Repeatedly cultured cancer cells showed the same tumorigenic ability as parental CLS1 cells and formed xenograft tumours in mice at a low cell number (100 cells; Supplementary Fig. 4b ). Figure 2: Lung CSCs maintain cancer stemness and high tumorigenicity when co-cultured with CAF feeders. ( a ) Our working hypothesis was that differentiated cancer cells would lose their cancer stemness after CAF removal. ( b ) RT Q–PCR analysis confirmed that the stemness markers Nanog and Oct3/4 were significantly reduced in CLS1 cells following passages without CAFs (from P1 to P14). The data represent the mean±s.d. ( N =3), and the different passages of CLS1 cells with CLS1/CAFs were tested by one-way analysis of variance with Tukey’s post hoc corrections. The data are representative of three independent biological experiments. ( c ) Immunofluorescence of Oct3/4 in CLS1 cells cultured with (CLS1/CAF) or without CAFs (CLS1) for 5 days. The arrow head shows glandular-type CLS1 cells that lost Oct3/4 staining after CAF removal. The nuclei were stained with DAPI. Retention assay of PKH26 positively stained cells among CLS1 cells. The cells were pre-stained with the PKH26 red fluorescent dye, and the cells were then co-cultured with or without CAFs for 1 week. Arrows mark the CLS1 cells that retained PKH26 fluorescence. Scale bar, 50 μm. ( d ) Spontaneous lung metastatic nodules of CLS1/CAF ( N =15 mice) and CLS1 ( N =10 mice) xenograft tumours (upper) were stained with haematoxylin and eosin (H&E; bottom). Scale bar, 100 μm. ( e ) IHC analysis for Oct3/4 and Nanog expression in a xenograft tumour (subcutaneous and spontaneous lung metastasis tumour) derived from injection of a CLS1 sphere co-cultured with CAFs. Scale bar, 50 μm. Full size image Table 1 Characteristics of CAFs isolated from NSCLC patients. Full size table Co-culture of CAFs with primary lung cancer cells (CL141 and CL152) as well as CLS1 cells can increase sphere-forming ability, larger sphere size ( Supplementary Fig. 5a ) and increased tumour-initiating frequency in xenografts compared with cancer cells subcultured without CAFs for an additional three passages ( Fig. 2d ). ALDH activity was also reduced after removing CAFs from the co-culture ( Supplementary Fig. 5b ). These results indicated that CAFs act as the key regulator of cancer stemness in primary lung cancer cells. Assessment of the cellular SP is another method for evaluating cancer stemness ability and drug resistance. CLS1 cells co-cultured with CAFs demonstrated a higher percentage of SP cells compared with other lung cancer cell lines, including CL1-5, A549, H522, H23, Hop62, H322M and EKVX ( Supplementary Fig. 5c ). The SP of CLS1 cells was significantly reduced after CAF removal ( Supplementary Fig. 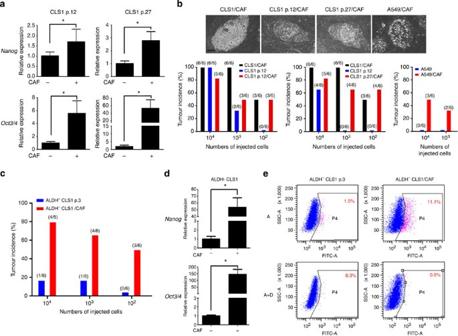Figure 3: Differentiated lung cancer cells can de-differentiate and re-acquire stem cell-like properties through re-co-culturing with CAFs. (a) RT Q–PCR analysis was performed to assess expression of the stemness markersNanogandOct3/4in CLS1 p.12 and CLS1 p.27 cells cultured with or without CAFs (N=3). (b) The incidence of mouse xenograft tumours from CLS1/CAF co-cultures (N=6 mice), differentiated CLS1 cells after 12 and 27 passages (p6 and p12;N=6 mice), A549 and CLS1 p.12/CAFs, CLS1 p.27/CAFs and A549/CAFs (N=6 mice) was determined following the subcutaneous injection of different cell numbers (1 × 104, 1 × 103and 1 × 102cells) into SCID mice. Scale bar, 200 μm. (c) The incidence of mouse xenograft tumours derived from sorted ALDH− CLS1 cells after three passages (p3;N=6 mice) and ALDH− CLS1/CAFs (N=6 mice) following subcutaneous injection into SCID mice at different cell numbers (1 × 104, 1 × 103and 1 × 102cells). (d) RT Q–PCR analysis was performed to assess expression of the stemness markersNanogandOct3/4in ALDH− CLS1 cells cultured with or without CAFs (N=3). (e) The ALDH activity of ALDH− CLS1 cells cultured with or without CAFs. ALDH activity was evaluated by staining with the ALDEFLUOR dye in the absence (upper) or presence (lower) of diethylaminobenzaldehyde (DEAB; an ALDH inhibitor) for 30 min at 37 °C and analysed by flow cytometry. The data represent the mean±s.d. and difference were tested by the Student’st-test; *P<0.05. The data are representative of at least three independent biological experiments. 5d ), and resistance to chemotherapeutic drugs (etoposide, docetaxel, vinorelbine ditartrate and cisplatin) was decreased ( Supplementary Table 3 ). CAF removal leads to ‘differentiation’ of CLS1 lung CSCs CLS1 cells co-cultured with CAFs (CLS1/CAF) maintained their cancer stemness phenotype. However, CLS1 cells became anchorage dependent and showed reduced Nanog and Oct3/4 expression after removal of the feeder cells. Some CLS1 cells even showed glandular differentiation concurrent with the loss of Oct3/4 ( Fig. 2c , arrow head) and different expression patterns of adenocarcinoma and squamous carcinoma markers (thyroid transcription factor (TTF)1, CK7, CK20, p63 and keratin 5/6) in different CLS1 single-cell clones (C1, 2, 3 and 4 clones; Supplementary Fig. 6a ). Immunohistochemistry (IHC) also showed differentiated cancer cells with different staining patterns (TTF1, CK7, CK20, p63 and keratin 5/6) in CLS1-formed xenografts ( Supplementary Fig. 6b ). These results indicated that CLS1 cells with stemness characteristics could be differentiated into different types of lung cancer cells expressing different adenocarcinoma and squamous cell carcinoma markers. Importantly, this pattern could be reversed by re-co-culturing with CAFs, leading to a downregulation of differentiation markers and a significant upregulation of Nanog and Oct3/4 ( Supplementary Fig. 7a,b ). CAFs promote stem cell-like properties in lung cancer cells Previously, we found that the removal of CAFs led to differentiation and loss of stemness characteristics among lung CSCs. In particular, we found that differentiated cancer cells (CLS1 p12, CLS1 p27 and A549 cells) could be de-differentiated by re-co-culturing with CAFs to regain cancer stem-like properties, with an increased expression of stemness markers ( Nanog and Oct3/4 ; Fig. 3a ) as well as the ability to form xenografts after the intradermal administration of as few as 100 cells ( Fig. 3b ). These data further support the notion that differentiated lung cancer cells could be induced to ‘de-differentiate.’ Next, CLS1 cells with negative ALDH activity (ALDH−) were sorted as the differentiated (non-CSC) population; then, these ALDH− CLS1 cells were co-cultured with CAFs to determine whether CAFs have the ability to promote tumorigenesis via an increase in cancer stemness. The results showed that the ALDH− population had very low tumorigenic ability in a xenograft model ( Fig. 3c ). Interestingly, these ALDH− CLS1 cells regained a high tumorigenic ability after re-co-culturing with CAFs; in particular, their cancer stemness properties were re-activated, and their expression of stemness markers increased ( Nanog and Oct3/4 increased 53.8- and 145.3-fold, respectively; ALDH activity increased 8.83-fold; tumour-initiating frequency increased from 1/7,917 to 1/91; Fig. 3c–e ). Figure 3: Differentiated lung cancer cells can de-differentiate and re-acquire stem cell-like properties through re-co-culturing with CAFs. ( a ) RT Q–PCR analysis was performed to assess expression of the stemness markers Nanog and Oct3/4 in CLS1 p.12 and CLS1 p.27 cells cultured with or without CAFs ( N =3). ( b ) The incidence of mouse xenograft tumours from CLS1/CAF co-cultures ( N =6 mice), differentiated CLS1 cells after 12 and 27 passages (p6 and p12; N =6 mice), A549 and CLS1 p.12/CAFs, CLS1 p.27/CAFs and A549/CAFs ( N =6 mice) was determined following the subcutaneous injection of different cell numbers (1 × 10 4 , 1 × 10 3 and 1 × 10 2 cells) into SCID mice. Scale bar, 200 μm. ( c ) The incidence of mouse xenograft tumours derived from sorted ALDH− CLS1 cells after three passages (p3; N =6 mice) and ALDH− CLS1/CAFs ( N =6 mice) following subcutaneous injection into SCID mice at different cell numbers (1 × 10 4 , 1 × 10 3 and 1 × 10 2 cells). ( d ) RT Q–PCR analysis was performed to assess expression of the stemness markers Nanog and Oct3/4 in ALDH− CLS1 cells cultured with or without CAFs ( N =3). ( e ) The ALDH activity of ALDH− CLS1 cells cultured with or without CAFs. ALDH activity was evaluated by staining with the ALDEFLUOR dye in the absence (upper) or presence (lower) of diethylaminobenzaldehyde (DEAB; an ALDH inhibitor) for 30 min at 37 °C and analysed by flow cytometry. The data represent the mean±s.d. and difference were tested by the Student’s t -test; * P <0.05. The data are representative of at least three independent biological experiments. Full size image According to these results, we suggest that the Oct3/4(+) and Nanog(+) CSC population can be maintained by CAF feeders but is reduced after CAF removal, and this population can also be re-programmed to regain stemness after re-co-culturing with CAFs ( Fig. 2a ). This CSC/CAF co-culture system therefore represents a good model to study how the microenvironment affects CSCs, particularly how the differentiation of tumorigenic CSCs into less tumorigenic cancer cells is affected by the tumour microenvironment [45] . Transcriptomic profiling reveals a stemness pathway in CSCs To discover cancer stemness-specific signalling pathways in lung CSCs, we analysed the gene expression profile of Oct3/4(+)/Nanog(+) CLS1 CSCs (CLS1/CAF) and compared this profile with that of CLS1-differentiated cancer cells cultured without feeder cells through different passages (CLS1 p3, p6 and p12; Supplementary Fig. 8a ). According to the transcriptome and MetaCore software analysis, stemness pathways related to IGF1R, EMT, phosphatidylinositol 3-kinase (PI3K), TGF-β, WNT and Hedgehog pathways, which regulate several stemness transcriptional factors (Oct3/4, Nanog and Sox2), were upregulated in the CLS1/CAF co-culture, whereas dramatically reduced following serial passage without CAFs ( Supplementary Fig. 8a,b ). Some of the pathways identified in these CLS1/CAF co-cultures, such as EMT, TGF-β and Hedgehog signalling, have been reported to be involved in maintaining cancer stemness [46] , [47] , [48] . For instance, EMT regulated by multiple epigenetic mechanisms is known to repress the expression of epithelial markers and to convert epithelial cells into aggressive, invasive tumour cells with stem cell properties [46] . These results indicated the presence of a complicated regulatory network for maintaining cancer stemness in lung CSCs ( Supplementary Fig. 8b ). Some of the key regulators identified, including TGFBR1 (TGF receptor 1), TCF21 (transcription factor 21), leukaemia inhibitory factor ( LIF ), LIF receptor ( LIFR ), early growth response 1 and SMAD2, were validated by quantitative (Q–PCR), showing a decreasing trend following serial passage without CAFs ( Supplementary Fig. 8c ). Interestingly, these stemness pathways may be triggered via extracellular signalling, indicating that paracrine and autocrine regulation may contribute to maintaining the CSC population in vivo . CAFs regulate cancer stemness through a paracrine network To better understand how CAFs contribute to maintaining lung cancer stemness, both the transcriptional regulation network and the cytokine network in/between CAF and CLS1 cells were studied. Interestingly, CAFs highly express several growth factors, including IGF-II , hepatocyte growth factor ( HGF ), LIF and stromal cell-derived factor 1 ( SDF1 ). Conversely, the receptors for these growth factor, including IGF1R , IGF2R , HGF receptor ( HGFR ), LIFR and C-X-C chemokine receptor type 4 ( CXCR4 ), as well as related signalling modulators such as IGF-binding proteins ( IGFBP s), were highly expressed in CLS1 cells ( Fig. 4a,b ). This observation suggested the presence of crosstalk and the existence of paracrine regulation between CAF and CLS1 cells. Most importantly, we found that conditioned medium obtained from the CLS1/CAF co-culture system could significantly upregulate Nanog expression in CLS1 cells ( Fig. 4c ). To explore this mechanism of paracrine regulation, the human chemokine and cytokine antibody array (Ray Biotech Inc., Norcross, GA), including 274 specific antibodies, was used, which demonstrated that a number of cytokines were relatively abundant in the CLS1/CAF co-culture medium ( Fig. 4d,e ). 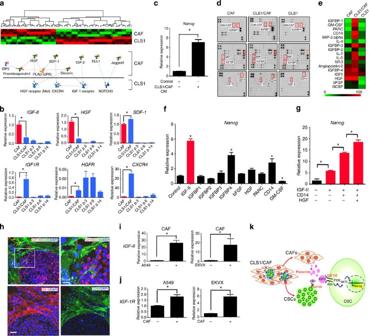Figure 4: Paracrine networks and the corresponding receptor pathways in CSC and CAF crosstalk. (a) Hierarchical clustering of differentially expressed genes in CSC (CLS1) cells cultured with or without CAFs. (b) RT Q–PCR validation of the paracrine regulatory pathway. CLS1 cells were derived from CLS1 spheres, dissociated to single cells and then subcultured without CAFs for different numbers of passages (p3, p6 and p14). CAFs served as the feeder cell control (N=3). (c) RT Q–PCR analysis of the stem cell markerNanogin CLS1 cells cultured in conditioned medium. The conditioned medium was collected from CLS1 cells co-cultured with CAFs (N=3). (d) Antibody arrays were used to examine the growth factors secreted by CAFs or the CLS1 cells cultured with or without CAFs in serum-free RPMI medium for 24 h. The arrays were scanned and quantified, and the levels were normalized to those of the positive controls. (e) The semiquantitative results of cytokine expression levels are represented as a heat map. (f) RT Q–PCR analysis of the stem cell markerNanogin CLS1 cells were treated with the following cytokines: IGF-II (10 ng ml−1); IGFBP1 (10 ng ml−1); IGFBP2 (10 ng ml−1); IGFBP3 (10 ng ml−1); IGFBP4 (100 ng ml−1); bFGF (10 ng ml−1); HGF (10 ng ml−1); PARC (pulomonary and activation-regulated chemokine) (10 ng ml−1); sCD14 (500 ng ml−1) and granulocyte-macrophage colony-stimulating factor (GM-CSF; 1 ng ml−1;N=3). (g) RT Q–PCR analysis of the stem cell markerNanogin CLS1 cells treated with IGF-II (10 ng ml−1) and combination of HGF (10 ng ml−1) and sCD14 (500 ng ml−1;N=3). (h) Immunofluorescence showing that IGF1R and IGF-II differentially localize in CLS1 cells and CAFs. IGF1R staining was observed in lung CSCs (red, upper panel). CD90-positive CAFs (green) showed staining for IGF-II (red, lower panel). The nuclei were stained with DAPI (blue;N=3). Scale bar, 50 μm. (i) RT Q–PCR analysis ofIGF-IIin CAFs obtained from patients and cultured with or without cancer cells (N=6 with A549 cells andN=9 with EKVX cells). (j) RT Q–PCR analysis ofIGF1Rin cancer cell (A549 or EKVX) cultured with or without CAFs obtained from patients (N=4 patients). (k) A hypothetical model showing the crosstalk between CSCs and CAFs that may contribute to cancer stemness. The data represent the mean±s.d. and were tested for significance using (b–c, i–j) the Student’st-test or (f–g) one-way analysis of variance with Tukey’spost hoccorrections; *P<0.05. The data are representative of at least three independent biological experiments, with three or more replicates in each experiment. Figure 4: Paracrine networks and the corresponding receptor pathways in CSC and CAF crosstalk. ( a ) Hierarchical clustering of differentially expressed genes in CSC (CLS1) cells cultured with or without CAFs. ( b ) RT Q–PCR validation of the paracrine regulatory pathway. CLS1 cells were derived from CLS1 spheres, dissociated to single cells and then subcultured without CAFs for different numbers of passages (p3, p6 and p14). CAFs served as the feeder cell control ( N =3). ( c ) RT Q–PCR analysis of the stem cell marker Nanog in CLS1 cells cultured in conditioned medium. The conditioned medium was collected from CLS1 cells co-cultured with CAFs ( N =3). ( d ) Antibody arrays were used to examine the growth factors secreted by CAFs or the CLS1 cells cultured with or without CAFs in serum-free RPMI medium for 24 h. The arrays were scanned and quantified, and the levels were normalized to those of the positive controls. ( e ) The semiquantitative results of cytokine expression levels are represented as a heat map. ( f ) RT Q–PCR analysis of the stem cell marker Nanog in CLS1 cells were treated with the following cytokines: IGF-II (10 ng ml −1 ); IGFBP1 (10 ng ml −1 ); IGFBP2 (10 ng ml −1 ); IGFBP3 (10 ng ml −1 ); IGFBP4 (100 ng ml −1 ); bFGF (10 ng ml −1 ); HGF (10 ng ml −1 ); PARC (pulomonary and activation-regulated chemokine) (10 ng ml −1 ); sCD14 (500 ng ml −1 ) and granulocyte-macrophage colony-stimulating factor (GM-CSF; 1 ng ml −1 ; N =3). ( g ) RT Q–PCR analysis of the stem cell marker Nanog in CLS1 cells treated with IGF-II (10 ng ml −1 ) and combination of HGF (10 ng ml −1 ) and sCD14 (500 ng ml −1 ; N =3). ( h ) Immunofluorescence showing that IGF1R and IGF-II differentially localize in CLS1 cells and CAFs. IGF1R staining was observed in lung CSCs (red, upper panel). CD90-positive CAFs (green) showed staining for IGF-II (red, lower panel). The nuclei were stained with DAPI (blue; N =3). Scale bar, 50 μm. ( i ) RT Q–PCR analysis of IGF-II in CAFs obtained from patients and cultured with or without cancer cells ( N =6 with A549 cells and N =9 with EKVX cells). ( j ) RT Q–PCR analysis of IGF1R in cancer cell (A549 or EKVX) cultured with or without CAFs obtained from patients ( N =4 patients). ( k ) A hypothetical model showing the crosstalk between CSCs and CAFs that may contribute to cancer stemness. The data represent the mean±s.d. and were tested for significance using ( b – c, i – j ) the Student’s t -test or ( f – g ) one-way analysis of variance with Tukey’s post hoc corrections; * P <0.05. The data are representative of at least three independent biological experiments, with three or more replicates in each experiment. Full size image Among these candidate cytokines identified, we found that IGF-II, soluble CD14 and HGF individually induced Nanog expression in CLS1 cells ( Fig. 4f ), with IGF-II showing the greatest effect. Interestingly, HGF and soluble CD14 synergistically increased the effects of IGF-II-induced Nanog expression by 20-fold in CLS1 cells ( Fig. 4g ). Importantly, we found that IGF did not act as an autocrine factor, as it does in hepatocellular carcinoma [49] ; instead, we showed the paracrine regulation of IGF-II from CAFs acting on the IGF1R dominantly expressed in lung CSCs (CLS1) as well as other IGF-response factors ( IGF2R , IGFBP1 and IGFBP2 ; Fig. 4b and Supplementary Fig. 9 ). Immunofluorescence staining further confirmed that IGF1R was abundantly expressed in lung CSCs, whereas IGF-II was predominantly expressed in CAFs ( Fig. 4h ). In addition, HGFR and CXCR4 messenger RNAs were expressed in CLS1 cells, whereas HGF and SDF1 were more highly expressed in CAFs ( Fig. 4a,b ). Furthermore, we hypothesized that the reciprocal interaction of genes induced in CAFs by co-culture with lung cancer cells is also important in regulating the cancer stemness niche. In fact, we found that several critical paracrine factors, including IGF-II , HGF and SDF-1 , are released from CAFs and may play important roles in maintaining cancer stemness ( Fig. 4b ). Moreover, these factors could be regulated by co-culture with cancer cells (CLS1, A549 and EKVX cells; Fig. 4i and Supplementary Fig. 10 ). Thus, we suggest that the cancer stemness niche could involve two-way communication between cancer cells and CAFs. CAFs support stemness through IGF-II/IGF1R/Nanog signalling To further evaluate whether IGF-II could be produced in all tumour-derived CAFs, isolated CAFs from different lung cancer patients were co-cultured with different lung cancer cells. Laser-captured feeder cells from different CAF samples showed higher expression levels of IGF-II ( N =6 with A549 cells and N =9 with EKVX cells; Fig. 4i ). Similarly, colony cells from cancer cells cultured with CAFs ( N =4) showed higher IGF1R expression levels ( Fig. 4j ). The characteristics of the 12 CAF samples isolated from patients are shown in Table 1 . We therefore propose a putative signalling crosstalk model involving paracrine interactions between CAFs and lung CSCs that contribute to cancer stemness ( Fig. 4k ). To further validate the roles of IGF-II signalling on cancer stemness in lung CSCs, several cancer stemness characteristics were examined in CLS1 and other lung cancer cell lines. We found that IGF-II increased the Nanog expression ( Fig. 5a ), and enlarged the sphere numbers and size ( Fig. 5b ), facilitated the number of Nanog-positive cells per colony through image-based high-content analysis (HCA; Supplementary Fig. 11a,b ) and increased the ALDEFLUOR-positive ratio ( Supplementary Fig. 12a,b ) in various lung cancer cells (CLS1/CAFs, A549, H1975 and EKVX). Western blotting further showed that IGF-II induced IGF1R and Akt phosphorylation and downstream Nanog expression in a time-dependent manner in primary lung cancer cells (CLS1, CL141 and CL152; Fig. 5c ). Moreover, the PI3K inhibitor LY294002 significantly reduced the number of Nanog-positive cells per colony in primary lung cancer cells (CLS1, CL141 and CL152) co-cultured with CAFs ( Supplementary Fig. 13a ). In addition, LY294002 could inhibit IGF-II-induced Akt-phosphorylation and Nanog expression ( Supplementary Fig. 13b ) and reduce the tumorigenicity of CLS1 cells (10 3 cells) in NOD/SCID mice ( Supplementary Fig. 13c ). Together, these results suggest that PI3K could be the intermediary component of the IGF-II/IGF1R/Nanog signalling pathway and that blocking PI3K signalling may thereby reduce IGF-II-regulated cancer stemness. 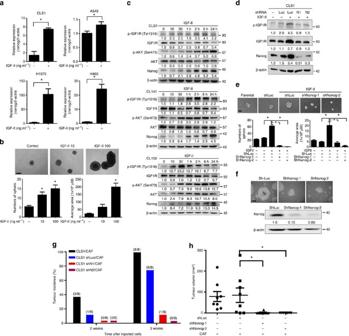Figure 5: The IGF-II/IGF1R/Nanog pathway is involved in microenvironmental paracrine signalling for maintaining the stemness of lung CSCs. (a) RT Q–PCR analysis of the stem cell markerNanogfor four different lung cancer cell lines (CLS1, A549, H1975 and H460) treated with IGF-II (100 ng ml−1;N=3). (b) The sphere-forming ability (lower panel) and morphology (upper panel) of CLS1 cells treated with IGF-II (10 and 100 ng ml−1) after culturing in MCDB201 medium with epidermal growth factor (EGF; 20 ng ml−1) and bFGF (20 ng ml−1) for 21 days. Scale bar, 100 μm. (c) Western blot analysis of IGF1R, AKT and Nanog expression in CLS1 cells treated with IGF-II (10 ng ml−1) and in primary cell lines (CL141 and CL152 cells) treated with IGF-II (100 ng ml−1) at the indicated time points (0, 10 and 30 min and 1, 2, 6 and 24 h). (d) Protein levels of Nanog-targeting short hairpin RNA (shRNA) Nanog (shN1 and shN2) or scrambled short interfering RNA (siRNA; shLuc) cells treated with IGF-II (10 ng ml−1) for 24 h were examined through immunoblotting. β-Actin was used as an internal control. (e) Sphere-forming ability (numbers of sphere,N=6; average area of sphere,N=10) and morphology of CLS1 cells treated with IGF-II (10 ng ml−1) and analysis of the specific knockdown of Nanog after culturing in MCDB201 medium with EGF (20 ng ml−1) and bFGF (20 ng ml−1) for 14 days. Scale bar, 50 μm. (f) Protein levels of Nanog in Nanog-targeted shRNA cells (shN1 and shN2) or scrambled siRNA (shLuc) cells were examined through immunoblotting. β-Actin was used as an internal control. Scale bar, 200 μm.(g) The incidence of xenograft tumours formed from CLS1/CAF cells with or without shRNA-mediated Nanog knockdown. The tumours were generated by the injection of 1,000 CLS1/CAF cells (N=8 mice). (h) The tumour volumes formed by CLS1/CAF cells with or without Nanog knockdown (N=8 mice). The data represent the mean±s.d. and were tested for significance by (a) the Student’st-test or (b–h) one-way analysis of variance with Tukey’spost hoccorrections; *P<0.05. The data are representative of three independent experiments, with three or more replicates in each experiment. Figure 5: The IGF-II/IGF1R/Nanog pathway is involved in microenvironmental paracrine signalling for maintaining the stemness of lung CSCs. ( a ) RT Q–PCR analysis of the stem cell marker Nanog for four different lung cancer cell lines (CLS1, A549, H1975 and H460) treated with IGF-II (100 ng ml −1 ; N =3). ( b ) The sphere-forming ability (lower panel) and morphology (upper panel) of CLS1 cells treated with IGF-II (10 and 100 ng ml −1 ) after culturing in MCDB201 medium with epidermal growth factor (EGF; 20 ng ml −1 ) and bFGF (20 ng ml −1 ) for 21 days. Scale bar, 100 μm. ( c ) Western blot analysis of IGF1R, AKT and Nanog expression in CLS1 cells treated with IGF-II (10 ng ml −1 ) and in primary cell lines (CL141 and CL152 cells) treated with IGF-II (100 ng ml −1 ) at the indicated time points (0, 10 and 30 min and 1, 2, 6 and 24 h). ( d ) Protein levels of Nanog-targeting short hairpin RNA (shRNA) Nanog (shN1 and shN2) or scrambled short interfering RNA (siRNA; shLuc) cells treated with IGF-II (10 ng ml −1 ) for 24 h were examined through immunoblotting. β-Actin was used as an internal control. ( e ) Sphere-forming ability (numbers of sphere, N =6; average area of sphere, N =10) and morphology of CLS1 cells treated with IGF-II (10 ng ml −1 ) and analysis of the specific knockdown of Nanog after culturing in MCDB201 medium with EGF (20 ng ml −1 ) and bFGF (20 ng ml −1 ) for 14 days. Scale bar, 50 μm. ( f ) Protein levels of Nanog in Nanog-targeted shRNA cells (shN1 and shN2) or scrambled siRNA (shLuc) cells were examined through immunoblotting. β-Actin was used as an internal control. Scale bar, 200 μm. ( g ) The incidence of xenograft tumours formed from CLS1/CAF cells with or without shRNA-mediated Nanog knockdown. The tumours were generated by the injection of 1,000 CLS1/CAF cells ( N =8 mice). ( h ) The tumour volumes formed by CLS1/CAF cells with or without Nanog knockdown ( N =8 mice). The data represent the mean±s.d. and were tested for significance by ( a ) the Student’s t -test or ( b – h ) one-way analysis of variance with Tukey’s post hoc corrections; * P <0.05. The data are representative of three independent experiments, with three or more replicates in each experiment. Full size image Furthermore, we found that IGF-II-regulated cancer stemness could be attenuated by the specific knockdown of Nanog. As shown in Fig. 5d , an short hairpin RNA against Nanog inhibited IGF-II-induced p-IGF1R and Nanog expression and reduced sphere-forming ability in vitro ( Fig. 5e,f ) and tumorigenicity in NOD/SCID mice ( Fig. 5g,h ), indicating the importance of Nanog in IGF-II-induced lung cancer stemness. Blockade of IGF1R signalling suppresses lung cancer stemness To further evaluate whether IGF-II signalling is a druggable pathway for anticancer therapy by targeting lung CSCs, specific IGF1R blockade strategies were used. Image-based HCA showed that the Nanog-positive cells in each colony were significantly inhibited in the presence of a specific IGF1R antibody or IGF1R inhibitors (picropodophyllin and AEW541) in lung cancer cell lines (A549, EKVX) and primary lung cancer cells (CLS1, CL141 and CL152; Fig. 6a and Supplementary Fig. 14a,b ). Using an IGF1R-blocking antibody (IGF1Rα Ab), we further confirmed that the sphere-forming ability of CLS1 cells was reduced following the blockade of IGF1R signalling ( Fig. 6b ); similar effects were observed in A549 and EKVX cells ( Supplementary Fig. 14c ). We also found that the ALDEFLUOR-positive ratio, which was substantially increased after IGF-II treatment, was blocked following the addition of IGF1Rα Ab in lung cancer cell lines (CLS1, A549, H1975 and EKVX; Fig. 6c ). Moreover, the IGF-II-mediated upregulation of Nanog expression, as well as IGF-II-induced IGF1R phosphorylation, Akt phosphorylation and downstream Nanog signalling in CLS1, CL141 and CL152 cells was inhibited when IGF1R signalling was blocked ( Fig. 6d,e ). Most importantly, the IGF1Rα Ab and inhibitor (AEW541) significantly reduced the tumorigenicity of CLS1 cells (10 3 cells) injected into NOD/SCID mice ( Fig. 6f and Supplementary Fig. 15 ), revealing that IGF-II signalling represents a potential anticancer target for lung CSCs. 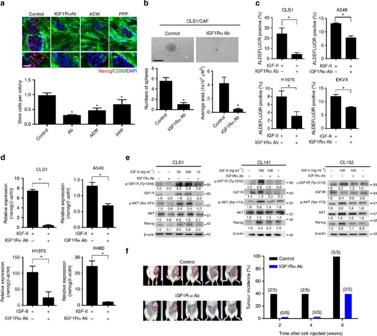Figure 6:The IGF-II/IGF1R signalling pathway as a target to suppress lung cancer stemness and tumorigenicity. (a) Nanog-positive stem cells per colony were analysed through image-based HCA. CLS1 cells were co-cultured with CAFs treated with or without an IGF1R-neutralizing antibody (IGF1Rα Ab; 1 μg ml−1) and an IGF signalling inhibitor (AEW541 and PPP (picropodophyllin) 1 μM ml−1;N=3). Scale bar, 50 μm. (b) The sphere-forming morphology and ability (numbers of sphere,N=6; average area of sphere,N=10) of the CLS1 were significantly reduced by treatment with IGF1Rα Ab (1 μg ml−1). Scale bar, 200 μm. (c) ALDH activity was examined using flow cytometry for four different lung cancer cell lines (CLS1, A549, H1975 and EKVX) treated with IGF-II (100 ng ml−1) or IGF-II in combination with IGF1Rα Ab (N=3). (d) RT Q–PCR analysis of the stem cell marker Nanog expressed in CLS1, A549, H1975 and H460 cells treated with IGF-II (100 ng ml−1) or IGF-II in combination with IGF1Rα Ab (N=3). (e) Western blot analysis of IGF1R-p/IGF1R, AKT-p/AKT and Nanog in CLS1 cells treated with IGF-II or IGF-II in combination with IGF1Rα Ab (1 μg ml−1) for 6 h (CLS1 cells) or 24 h (CL141 and CL152 cells). (f) The incidence of xenograft tumours formed from CLS1/CAF cells was reduced following treatment with 1 μg ml−1IGF1Rα Ab. The tumours were generated by the injection of 1,000 CLS1/CAF cells (N=5 mice). The tumour-forming ability of CLS1/CAF cells was inhibited by IGF1Rα Ab (1 μg ml−1) treatment (N=5 mice; 100% (5/5) in control versus 40% (2/5) in IGF1Rα Ab-treated group). The data represent the mean±s.d. and were tested for significance by (a) one-way analysis of variance with Turkey’spost hoccorrections or (b–d) the Student’st-test; *P<0.05. The data are representative of three independent experiments, with three or more replicates in each experiment. Figure 6: The IGF-II/IGF1R signalling pathway as a target to suppress lung cancer stemness and tumorigenicity . ( a ) Nanog-positive stem cells per colony were analysed through image-based HCA. CLS1 cells were co-cultured with CAFs treated with or without an IGF1R-neutralizing antibody (IGF1Rα Ab; 1 μg ml −1 ) and an IGF signalling inhibitor (AEW541 and PPP (picropodophyllin) 1 μM ml −1 ; N =3). Scale bar, 50 μm. ( b ) The sphere-forming morphology and ability (numbers of sphere, N =6; average area of sphere, N =10) of the CLS1 were significantly reduced by treatment with IGF1Rα Ab (1 μg ml −1 ). Scale bar, 200 μm. ( c ) ALDH activity was examined using flow cytometry for four different lung cancer cell lines (CLS1, A549, H1975 and EKVX) treated with IGF-II (100 ng ml −1 ) or IGF-II in combination with IGF1Rα Ab ( N =3). ( d ) RT Q–PCR analysis of the stem cell marker Nanog expressed in CLS1, A549, H1975 and H460 cells treated with IGF-II (100 ng ml −1 ) or IGF-II in combination with IGF1Rα Ab ( N =3). ( e ) Western blot analysis of IGF1R-p/IGF1R, AKT-p/AKT and Nanog in CLS1 cells treated with IGF-II or IGF-II in combination with IGF1Rα Ab (1 μg ml −1 ) for 6 h (CLS1 cells) or 24 h (CL141 and CL152 cells). ( f ) The incidence of xenograft tumours formed from CLS1/CAF cells was reduced following treatment with 1 μg ml −1 IGF1Rα Ab. The tumours were generated by the injection of 1,000 CLS1/CAF cells ( N =5 mice). The tumour-forming ability of CLS1/CAF cells was inhibited by IGF1Rα Ab (1 μg ml −1 ) treatment ( N =5 mice; 100% (5/5) in control versus 40% (2/5) in IGF1Rα Ab-treated group). The data represent the mean±s.d. and were tested for significance by ( a ) one-way analysis of variance with Turkey’s post hoc corrections or ( b – d ) the Student’s t -test; * P <0.05. The data are representative of three independent experiments, with three or more replicates in each experiment. Full size image IGF-II-IGF1R/Nanog levels correlate with poor prognosis We previously demonstrated that CAFs act as ‘feeders’ that secrete IGF-II and act on IGF1R in lung cancer cells, driving stemness pathways and maintaining the cancer stemness characteristics. To examine the clinical relevance and importance of IGF-II/IGF1R/Nanog paracrine regulation in the early stages of tumorigenesis, tumour specimens from 80 patients with stage I NSCLC who had not received preoperative chemo- or radiotherapy were collected, and serial sections of each specimen were stained with antibodies against IGF-II, IGF1R and Nanog via IHC. The clinical characteristics of these patients are summarized in Supplementary Tables 4–6 . The levels of IGF-II in CAFs and of IGF1R/Nanog in tumour cells were scored and dichotomized to high (score ≥median risk score) or low (score<median risk score) IGF-II, IGF1R and Nanog protein expression categories. A tree diagram was created to display the conditional probabilities of IGF-II, IGF1R and Nanog expression, as shown in Fig. 7a . These results indicated that 72% patients with high IGF-II and high IGF1R expression levels also demonstrated high Nanog expression levels, whereas 80.6% patients with low expression levels of IGF-II and IGF1R demonstrated lower Nanog expression levels. Next, serial sections of each specimen were stained with antibodies against IGF-II in CAFs and against IGF1R and Nanog in tumour cells, as shown in Fig. 7b . These results indicated that patients with high-level of IGF-II in CAFs and IGF1R or Nanog in tumour cells demonstrated significantly poorer overall survival ( P <0.0001, the Kaplan–Meier analysis; Fig. 7c ) and relapse-free survival ( P <0.0001, the Kaplan–Meier analysis; Fig. 7d ) compared with patients with low-level expression. 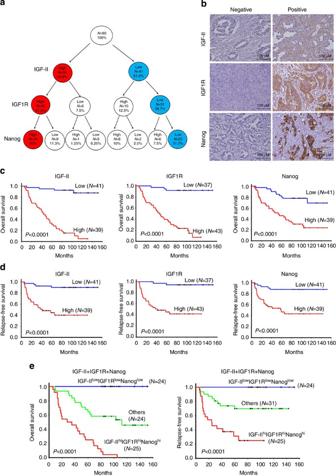Figure 7: Clinical significance of IGF-II in CAFs and IGF1R as well as Nanog in cancer cells for stage I NSCLC patients. (a) A tree diagram showing the proportions of patients with high and low IGF-II expression levels in CAFs and IGF1R/Nanog expression in tumour cells. (b) IHC staining of IGF-II in CAFs and IGF1R/Nanog in cancer cells from serial dissections of primary tumour specimens obtained from a clinical cohort of 80 patients with stage I NSCLC who underwent surgical resections. The images were obtained from different patients with low (score <median risk score) and high (score ≥median risk score) expression of IGF-II in CAFs and IGF1R/Nanog in cancer cells (original magnification, × 100). (c,d) The patients were designated as having high or low IGF-II, IGF1R and Nanog expression (cutoff value=median risk score). The results showed a significant difference in the Kaplan–Meier estimates of overall (c) and relapse-free (d) survival between the high and low expression groups.Pvalues were obtained from two-sided log-rank tests. (e) By combining the expression levels of IGF-II in CAFs and IGF1R/Nanog in cancer cells, the patients were divided into three groups: a high IGF-II/high IGF1R/high Nanog group, a low IGF-II/low IGF1R/low Nanog group and others. The results showed a significant difference in Kaplan–Meier estimates of overall and relapse-free survival.Pvalues were obtained from two-sided log-rank tests. Figure 7: Clinical significance of IGF-II in CAFs and IGF1R as well as Nanog in cancer cells for stage I NSCLC patients. ( a ) A tree diagram showing the proportions of patients with high and low IGF-II expression levels in CAFs and IGF1R/Nanog expression in tumour cells. ( b ) IHC staining of IGF-II in CAFs and IGF1R/Nanog in cancer cells from serial dissections of primary tumour specimens obtained from a clinical cohort of 80 patients with stage I NSCLC who underwent surgical resections. The images were obtained from different patients with low (score <median risk score) and high (score ≥median risk score) expression of IGF-II in CAFs and IGF1R/Nanog in cancer cells (original magnification, × 100). ( c , d ) The patients were designated as having high or low IGF-II, IGF1R and Nanog expression (cutoff value=median risk score). The results showed a significant difference in the Kaplan–Meier estimates of overall ( c ) and relapse-free ( d ) survival between the high and low expression groups. P values were obtained from two-sided log-rank tests. ( e ) By combining the expression levels of IGF-II in CAFs and IGF1R/Nanog in cancer cells, the patients were divided into three groups: a high IGF-II/high IGF1R/high Nanog group, a low IGF-II/low IGF1R/low Nanog group and others. The results showed a significant difference in Kaplan–Meier estimates of overall and relapse-free survival. P values were obtained from two-sided log-rank tests. Full size image Multivariable Cox proportional hazards regression analyses were used to evaluate the associations of various independent prognostic factors with patient survival ( Table 2 ). Our results revealed that the independent prognostic factors included IGF-II expression (hazard ratio (HR)=19.15, 95% confidence interval (CI)=6.32–58.00; P <0.0001, Cox proportional hazards regression analysis), IGF1R expression (HR=15.80, 95% CI=5.85–65.96; P <0.0001, Cox proportional hazards regression analysis) and Nanog expression (HR=4.84, 95% CI=2.17–10.80; P =0.0001, Cox proportional hazards regression analysis). The independent prognostic factors associated with metastasis were IGF-II expression (HR=7.37, 95% CI=2.43–22.35; P =0.0004, Cox proportional hazards regression analysis), IGF1R expression (HR=13.29, 95% CI=3.09–57.23; P =0.0005, Cox proportional hazards regression analysis) and Nanog expression (HR=7.59, 95% CI=2.67–21.62; P =0.0001, Cox proportional hazards regression analysis; Supplementary Table 7 ). Analysis of the combined effect of both ligand and receptor on patient prognoses revealed that patients with high-level expression of IGF-II in CAFs and high-level expression of IGF1R and Nanog in tumour cells demonstrated the worst overall (IGF-II+IGF1R+Nanog, P <0.0001, the Kaplan–Meier analysis; Fig. 7e ; HR=8.37, 95% CI=33.84–18.26; P <0.0001, Cox proportional hazards regression analysis; Table 1 ) and relapse-free survival (IGF-II+IGF1R+Nanog, P <0.0001, the Kaplan–Meier analysis; Fig. 7e ; HR=5.02, 95% CI=2.41–10.47; P <0.0001, Cox proportional hazards regression analysis; Supplementary Table 7 ) compared with those with low-level expression of IGF-II in CAFs and low-level expression of IGF1R and Nanog in tumour cells. These results further demonstrate that IGF-II, IGF1R and Nanog paracrine signalling may provide a novel prognostic index for predicting metastasis ( P <0.0001, Cox proportional hazards regression analysis) and overall survival ( P <0.0001, Cox proportional hazards regression analysis) in early-stage NSCLC patients ( Table 2 and Supplementary Table 7 ). Table 2 Multivariate Cox proportional hazards regression analysis with covariates. Full size table One key factor that hinders CSC research is the lack of a powerful culture system to support CSC growth while preserving stemness. Moreover, traditional embryonic stem cell culture systems that use fibroblasts as feeder cells have not yet successfully translated into a working model for CSC research. Here, for the first time, we established primary cultures of lung CSCs from lung cancer patients. Importantly, lung CSCs could be subcultured while maintaining the characteristics of cancer stemness using CAFs as feeder cells. In this study, we showed that CAFs, but not NFs, supported CSC growth. These CSCs isolated from primary cultures of lung tumours and cancer cell lines maintained their ability to express stemness markers and generate tumours in mouse xenografts at low cell numbers (<100 cells), and CAFs were essential for maintaining this stemness phenotype. Without the support of CAF feeder cells, lung CSCs differentiated into cancer cells. Interestingly, the addition of CAFs as niche cells could facilitate the conversion of differentiated tumour cells to CSC state through paracrine activation of EMT/MNNG HOS transforming gene (MET) [39] , WNT, Notch and Hedgehog signalling [39] . Most importantly, we found that CAFs could regulate CSC growth in a paracrine manner by overexpression of growth factors such as IGF-II , HGF and SDF1 and by inducing expression of the corresponding receptors in CSCs, including IGF1R , IGF2R , HGFR and CXCR4 . Moreover, the CAFs secreted IGF-II to stimulate the IGF1R on CSCs and thus activate the IGF-II/IGF1R/Nanog signalling pathway, which maintained lung cancer stemness in vitro and in vivo . In summary, our data support the CSC model and suggest the presence of autocrine regulation [50] ; however, there were paracrine interactions between CAFs and CSCs that were crucial for maintaining the cancer stemness niche of lung CSCs ( Fig. 8 ). 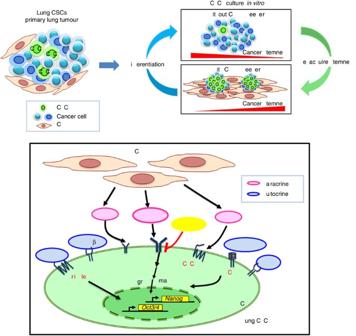Figure 8: A schematic illustration of the crosstalk between CAFs and lung CSCs. CAFs secrete IGF-II, which activates IGF1R/Nanog in lung CSCs through IGF1R signalling and Akt phosphorylation. On triggering the paracrine IGF-II/IGF1R pathway, other autocrine (LIF and LIFR; TGF-β and TGFBR1; WNT and Frizzled receptor) and paracrine (HGF and HGFR/c-MET; SDF-1 and CXCR4) signalling between CAFs and CSCs may contribute synergistically to the maintenance of lung CSC stemness. Figure 8: A schematic illustration of the crosstalk between CAFs and lung CSCs. CAFs secrete IGF-II, which activates IGF1R/Nanog in lung CSCs through IGF1R signalling and Akt phosphorylation. On triggering the paracrine IGF-II/IGF1R pathway, other autocrine (LIF and LIFR; TGF-β and TGFBR1; WNT and Frizzled receptor) and paracrine (HGF and HGFR/c-MET; SDF-1 and CXCR4) signalling between CAFs and CSCs may contribute synergistically to the maintenance of lung CSC stemness. Full size image Importantly, using CAF feeder cells, the CSCs could be subcultured while retaining their cancer stemness characteristics. The present study compared CAFs with paired NFs from different patients, and we found that CAFs, but not NFs, stimulated the sphere-forming ability of CSCs and led to the expression of stemness markers in lung cancer cell lines, indicating that CAFs supported CSC growth in vitro . Previously described strategies for isolating CSCs include sorting CSCs from the tumour bulk using specific markers or by forming mamospheres on ultra-low adherent plates [22] , [23] . However, these methods do not allow for the maintenance or subculturing of CSCs in vitro . We found that using CAFs as feeder cells, CSCs could be subcultured while retaining their cancer stemness, and this concept is similar to the ability of mouse embryonic fibroblasts to maintain the stemness of human embryonic stem cells [26] , [50] . On the basis of this concept, we suggest a new model for culturing lung CSCs involving the use of CAFs obtained from cancer patients as feeder cells to overcome the current difficulty of maintaining cancer stemness in vitro . This method supports long-term lung CSC growth and subculturing while maintaining the cancer stemness phenotype, and this platform should prove useful for drug screening and development of novel therapeutic strategies targeting CSCs or the stemness niche. Previous studies have revealed the types of cells involved in the tumour microenvironment, including infiltrating immune cells (for example, tumour-associated macrophages), and CAFs are crucial for driving the hallmarks of cancer, including tumorigenesis, angiogenesis and metastasis [51] , [52] . However, it remains less well understood how the tumour microenvironment supports cancer stemness [52] , [53] . ES cell research has shown that feeder cells are essential for supporting stem cell growth and the inhibition of differentiation through the secretion of certain factors (for example, TGF-β1, LIF and basic fibroblast growth factor (bFGF)) [54] that activate important signalling (WNT, Notch, Hedgehog and EMT signalling). Our data demonstrate that CAFs (HGF, IGF-II, SDF-1, bFGF, WNT and oncostatin M) regulate CSC-like characteristics in a paracrine manner through the counterpart receptor/signalling components (EMT, TGF-β, WNT, Notch and Hedgehog) and stemness factors (Oct3/4, Sox2 and Nanog) in lung CSCs. Moreover, we confirmed the importance of the IGF-II/IGF1R/Nanog pathway in regulating lung CSC growth, predominantly in a paracrine manner in the tumour microenvironment, and in supporting lung cancer stemness. Through the interaction between lung CSCs and CAFs, lung CSCs could stimulate CAFs to produce IGF-II, which is important for triggering IGF1R signalling in CSCs. We further addressed the two-way paracrine communication between CSCs and CAFs and its role in promoting cancer stemness, and the results indicated that CAFs secreted IGF-II, HGF and SDF-1. These factors may play important roles in maintaining cancer stemness and were upregulated following co-culture with CSCs or cancer cells. Although the detailed mechanisms remain unclear, our data suggest that cytokines, including bFGF, HGF, IGFBP2, granulocyte-macrophage colony-stimulating factor and pulmonary and activation-regulated chemokine (PARC), which were abundant in CSC-conditioned medium, may be released by CAFs after the induction of IGF-II expression. Additional evidence from previous studies indicates that bFGF and TGF-β released from cancer cells may be involved in fibroblast activation [31] , [55] , and our findings indicate that the cancer stemness niche may share similar paracrine loops as those regulating human embryonic stem cells [56] . Furthermore, our data revealed two-way communication between cancer cells and CAFs. The regulation of CAFs in terms of IGF-II secretion could be upregulated by lung cancer cells or CSCs through bFGF and other cytokines, whereas the IGF-II/IGF1R axis promoted Nanog expression in cancer cells. A positive feedback loop may therefore exist, leading to increased IGF1R expression in CSCs and maintenance of CSC stemness [49] . This evidence supports the role of cancer–stroma interactions and the importance of the tumour microenvironment in regulating cancer stemness. Our data further indicated that blockade of IGF-II/IGF1R/Akt/Nanog signalling could reduce cancer stemness in CSCs, suggesting the potential clinical application of targeted therapy using an IGF1R inhibitor for lung CSCs. Recently, many new therapeutic strategies have been designed to target and eliminate CSCs; however, the tumour microenvironment has been suggested to play a dominant role in determining the malignant characteristics of CSCs [57] . It is particularly important to determine whether the ‘de-differentiation’ of non-tumorigenic cancer cells towards CSCs can occur in certain niches. Previous studies have suggested that cell plasticity and de-differentiation in normal somatic cells could be controlled by environmental factors or artificial transduction with the right factors [58] , [59] . Recently, tumour microenvironment stromal cells have been shown to induce the de-differentiation of intestinal epithelial cells that acquire tumour-initiating capacity during intestinal tumorigenesis [29] . In this study, we found that differentiated cancer cells (CLS1 p12, CLS1 p27 and A549 cells) and the non-cancerous stem cell population (ALDH− CLS1 cells) might be possibly de-differentiated through co-culture with CAFs to regain CSC-like properties and re-expression of stemness markers (Nanog and Oct3/4). However, our experiments still could not exclude the possibility of selection and expansion of a small population of CSC by co-culture with CAFs and the possibility that CAFs might facilitate the conversion of CSC’s states that is, EMT/MET rather than de-differentiation. Since the CSC states might express different markers, this could also be consistent with our results. Our finding provides evidence that de-differentiation of differentiated cancer cells may occur under the influence of the tumour microenvironment, that is, CAFs. Thus, the direct targeting of CSCs may not be sufficient to cure cancer; instead, tumour microenvironmental factors, such as the paracrine signalling loops between CAFs and CSCs, could represent the basis of new, innovative treatments targeting the CSC niche. Furthermore, we validated whether IGF-II/IGF1R paracrine and stemness marker Nanog could serve as novel prognostic markers in stage I NSCLC patients. Previously, most prognostic factor studies focused on cancer cells rather than on CAFs; only an 11-gene prognostic CAF signature has been reported to be associated with NSCLC patient survival [60] . However, the clinical impact of paracrine regulation between CAFs and CSCs has not been well studied. For the first time, we performed IHC staining to clearly distinguish the levels of IGF-II in CAFs and IGF1R/Nanog in cancer cells as important prognostic markers for early-stage lung cancer patients. In fact, the IGF-II levels in CAFs individually or in combination with the IGF1R and Nanog levels in cancer cells strongly correlated with the overall and relapse-free survivals. We conclude that IGF-II/IGF1R/Nanog paracrine signalling on tumour progression could serve as a prognostic marker for early-stage lung cancer. In conclusion, our approach provides new insights into the crosstalk between the tumour microenvironment and CSCs. The CLS1/CAF co-culture model may represent a new platform for anticancer drug screening to derive compounds targeting CSCs and tumour-associated stromal cells. Moreover, the finding that CAFs regulate CSCs in a paracrine manner through the IGF-II/IGF1R/Nanog pathway may provide new potential targets for anticancer therapy. Lung cancer cell lines The human NSCLC cell lines NCI-A549, NCI-H460, H1975 and NCI-EKVX were obtained from the National Cancer Institute (National Institutes of Health, Bethesda, MD, USA) or the American Type Culture Collection (Manassas, VA, USA). We also established human lung cancer cell lines (CL25, CL83, CL141 and CL152) using primary cultures from lung cancer patients with adenocarcinomas. The cells were cultured in RPMI 1640 medium supplemented with 10% fetal bovine serum at 37 °C under a humidified atmosphere consisting of 20% O 2 and 5% CO 2 . Primary cultures of lung cells Human lung CSCs and CAFs were harvested from freshly resected lung tumour tissues from lung cancer patients who underwent surgical resection at the National Taiwan University Hospital ( Supplementary Data and Table 2 ). Tumours and paired normal tissues were harvested within 30 min after resection to isolate primary lung CSC, CAF and NF cultures using a modified protocol [60] , [61] . Lung CSCs were isolated from cancer-associated regions of resected tissues from NSCLC patients and were cultured and maintained with feeder cells, that is, stromal fibroblasts. The samples were procured and utilized according to approved IRB protocols for research on human subjects (NTUH IRB201103028RC: Lung cancer stem cells: marker identification and clinical applications—To isolate cancer stem cell from lung cancer patient), National Taiwan University Hospital (NTUH). Written informed consent was obtained from all patients. Non-cancer-associated stromal was sampled by a pathologist at least 5 cm away from neoplastic lesions (under sterile conditions) within 30 min after resection, as determined by gross examination at the time of surgical excision and subsequent histological analysis. The tissues were processed based on a previously described protocol with modifications [62] . In brief, the tissues were minced and incubated for 6–12 h in the presence of deoxyribonuclease 1 (1 mg ml −1 ; Bioshop) and protease (1 mg ml −1 ; Sigma) in S-MEM medium (GIBCO, Gibco BRL Life technologies) at 4 °C. After digestion, cell clumps were sieved through a 40-μm cell strainer (Falcon) to obtain single-cell suspensions. The collected cells were cultured at different cell densities (5 × 10 5 ) in a 24-well plate with the modified culture conditions in RPMI 1640 with 10% fetal bovine serum at 37 °C in a humidified atmosphere containing 20% O 2 and 5% CO 2 . After 30 days of culture, sphere-like colonies could be identified with the surrounding stroma cells. Subculturing of sphere-like cells was performed as previously described with some modifications [62] . The spheres were collected through gentle centrifugation (58 g , 800 r.p.m.) after 7–10 days and dissociated enzymatically (10 min in 0.05% trypsin, 0.53 mM EDTA 4Na; Invitrogen) and mechanically using a fire-polished Pasteur pipette. The cells obtained from dissociation were passaged through a 40-μm sieve and analysed microscopically for single-cell status. The cells, at a density of 5,000 viable cells ml −1 , were plated in plates pre-seeded with stromal cells as feeders (5 × 10 5 cells per well). For the single cell per well clone experiments, the cells were plated in 96-well plates using a cell sorter during fluorescence activated cell sorting (FACS Ariel), and the wells had been pre-seeded with feeder cells (2,000 cells per well). Subculturing of lung CSCs was performed as previously described with some modifications [62] . In brief, spheres were collected through gentle centrifugation (58 g , 800 r.p.m. ), enzymatic digestion (10 min with 0.25% trypsin, 1 mM EDTA; Invitrogen) and mechanic disruption. The lung CSCs obtained from this dissociation were passaged through a 100-μm strainer, and the sieved cells were analysed microscopically. The single cells, at a density of 5,000 viable cells ml −1 , were plated on 10-cm dishes pre-seeded with CAF feeder cells (5 × 10 5 cells per well). Colony purification using the Cyntellect LEAP system Cancer cells were dissociated to single cells using trypsin in an EDTA-containing solution, and the single-cell suspension (500 viable cells per well) was added to C-lect six-well plates pre-seeded with stromal cells (5 × 10 4 cells per well). After colony formation, individual cells were purified using the LEAP system (Cyntellect). The LEAP Stem Cell Colony Purification Application Guide was followed. The plate was loaded into the LEAP instrument and processed using the colony purification application protocol. Image processing and gating of the colony purification region was performed with square shapes. The LEAP system displayed images of the selected cells for preview. Cell ablation was individually targeted using a green laser. After LEAP processing, the cultured cells were removed from the well with trypsin and cultured using standard cell culturing conditions. Real-time RT Q–PCR The expression level of stemness-related genes and validation of the Affymetrix microarray data for CAF, CLS1/CAF and CLS1 were performed through real-time reverse transcriptase (RT) Q–PCR using an ABI Prism 7900 Sequencer (Applied Biosystems). The primers were designed using Primer Express 3.0 (Applied Biosystems; Supplementary Table 8 ). TATA box-binding protein (TBP) and β-actin were used as internal controls. The expression levels were normalized to TBP and defined as −ΔCT=−[CT target −CT TBP ]. The relative expression ratio was calculated as the fold change relative to the control (2 −ΔΔCT ). The experiments were performed in triplicate. Immunofluorescence microscopy Cells were fixed with 4% paraformaldehyde in PBS at room temperature. A standard immunofluorescence protocol was followed [63] . Blocking and hybridization were performed in 3% (wt/vol) BSA in PBS. Monoclonal antibodies targeting Nanog (ReproCELL; 1:300) and Oct3/4 (H-134; Santa Cruz; 1:100), as well as CD90 fluorescein isothiocyanate (FITC)-conjugated (5E10; BD Pharmingen; 1:100), cytokeratin-7 (Dako; 1:50), cytokeratin-20 (Dako; 1:25), keratin 5/6 (Thermo; 1:10) and TTF1 (Dako) antibodies were used. The stained cells were examined using an Axiovert 200 microscope (Carl Zeiss, Göttingen, Germany), a confocal laser scanning microscope (C1si, Nikon, Japan) with MetaXpress (Molecular Devices) or flow cytometry (FACSAria, Becton Dickinson). Image-based high-content assay Lung CSCs or cancer cells (200 cells per well) were added to 96-well plates pre-seeded with CAFs (2,000 cells per well) and allowed to attach to the plates overnight. After different treatments, the cells were processed following the immunofluorescence protocol with the Nanog (ReproCELL; 1:300) primary antibody (as the cancer stem cell marker) and the mouse anti-human CD90 FITC-conjugated (5E10; BD Pharmingen; 1:100) antibody (as the CAF marker) overnight at 4 °C. Next, the primary antibodies were incubated with the tetramethyl rhodamine iso-thiocyanate (TRITC)-conjugated secondary antibody (goat anti-rabbit IgG (H+L) conjugate; Invitrogen) for 2 h at room temperature. The nuclei were counterstained with Hoechst 33342 dye (Invitrogen). To determine the background fluorescence level of the secondary antibody, each plate included control wells containing only the secondary antibody (stained with the Hoechst 33342 dye). Images of the stained cells were acquired using the automated fluorescence microscopy platform. Image acquisition and analysis The stained cells were imaged using the HCA platform with a × 4 objective. Twelve fields per well for each wavelength were captured and montaged for further image analysis. The images were analysed using the MetaXpress software (Molecular Devices). First, the cancer cell nuclei (cells without FITC staining, CD90−) were identified using multi-wavelength cell scoring. The segmented cancer cell nuclei were dilated and smoothed using morphology filters to create a cell cluster mask. Cell clusters greater than 10,000 μm 2 were defined as cancer cell colonies. Finally, the TRITC-stained cell count and the total cell count were determined. The stemness of each colony was calculated as the ratio of Nanog-positive (TRITC-stained) cells to total cells. The colony density was defined as the total cell count divided by the colony area. PKH26 retention assay Lung CSCs (10 6 cells per 100 μl) were labelled with 2 μM PKH26 red (Sigma) and incubated for 5 min at room temperature [21] . The labelled cells were washed three times with culture medium. The labelled cells were co-cultured with or without CAFs for 1 week. Distinctly red fluorescent, stained cells were monitored using fluorescence microscopy. Ultra-low sphere-forming assay An ultra-low sphere-forming assay was performed as previously described [62] and modified as the following procedures. A single-cell suspension of lung CSCs in MCDB201 serum-free medium (Invitrogen) supplemented with 20 ng ml −1 epidermal growth factor (Sigma) and 20 ng ml −1 bFGF (Invitrogen) was seeded in ultra-low adherent 24-well plates (Corning, Corning, NY, USA; 200 viable cells per well). The medium was supplemented with fresh growth factors twice weekly. After 3 weeks, the spheres were examined under the Axiovert 200 microscope. SP analysis Hoechst staining was performed as previously described [64] and modified as the following procedures. The cells were suspended at a density of 1 × 10 6 cells ml −1 in pre-warmed PBS (Invitrogen), and Hoechst 33342 dye (Invitrogen) was added at a final concentration of 5 μg ml −1 in the presence or absence of reserpine (50 μM; Sigma). The cells were incubated at 37 °C for 120 min with intermittent shaking, and at the end of the incubation, the cells were washed with PBS, centrifuged at 4 °C and resuspended in PBS. Propidium iodide (2 μg ml −1 ; Invitrogen) was added to gate viable cells. The suspension was then filtered through a 40-μM cell strainer to obtain a single-cell suspension before cell sorting. Analysis and sorting were performed using the FACSAria instrument (Becton Dickinson). The Hoechst 33342 dye was excited at 375 nm, and the fluorescence was analysed by dual-wavelength detection (blue, 450/20; red, 670LP). ALDEFLUOR assay ALDH activity of cells was measured using the ALDEFLUOR assay kit (StemCell Technologies) based on the manufacturer’s protocol and a previous report [63] . After different treatments, the cells were suspended in the ALDEFLUOR assay buffer containing the ALDH substrate BODIPY-aminoacetaldehyde (1 mM per 1 × 10 6 cells, incubated for 30 min at 37 °C). As a negative control, the cell sample was treated with diethylaminobenzaldehyde, a specific ALDH inhibitor. Non-viable cells were identified by propidium iodide staining and analysis using the FACSAria instrument (Becton Dickinson). Drug resistance assay An MTT [3-(4,5-dimethylthiazolyl-2)-2,5-diphenyltetrazolium bromide] (Sigma) assay was performed to determine cell proliferation. In brief, CLS1/CAF and CLS1 cells were added to 96-well plates at a density of 5 × 10 3 cells per well. After incubating for 24 h, the cells were serum starved overnight. The cells were then treated with different concentrations (0–50 μM) of the drugs docetaxel, cisplatin, etoposide and vinorelbine for 48 h. After 48 h, the culture medium containing 0.5 mg ml −1 MTT was added to each well. After 1.5 h of incubation, the medium was removed and dimethylsulphoxide was added to the plates. The colour intensity of the solubilized formazan was measured at 570 nm in an enzyme-linked immunosorbent assay plate reader (Vector3; Perkin-Elmer, USA). Xenograft tumour formation in SCID mice All procedures involving mice were approved by the Animal Care and Use Committee of the National Taiwan University. Six-week-old male SCID mice were used for the subcutaneous injection of lung cancer cells or CSCs in low doses (10 6 , 10 5 , 10 4 , 10 3 or 10 2 viable cells in 100 μl of Hank’s balanced salt solution mixed in Matrigel). The mice were monitored for 8 weeks, and the incidence of tumour formation and metastasis was examined. The tumour sections were stained with haematoxylin and eosin and analysed by IHC using antibodies targeting Nanog (ReproCELL), Oct3/4 (Santa Cruz; H-134) and vimentin (NCL-L-VIM-V9). The staining was visualized using an Ultra Vision detection system with an horseradish peroxidase (HPR) polymer (Dako) and the diaminobenzidine chromogen (Dako) followed by counterstaining with haematoxylin. Gene expression profiling and pathway analysis The gene expression profiling map of CAF, CLS1/CAF and CLS1 was obtained using the Affymetrix GeneChip system (Affymetrix Inc., Santa Clara, CA, USA) according to the manufacturer’s protocol. Gene expression profiling was performed using the Affymetrix GeneChip system (Affymetrix Inc.) according to the manufacturer’s protocol. The array data were processed by the National Taiwan University Microarray Core Facility for Genomic Medicine. In brief, total RNA isolated from CAFs, lung CSCs and cancer cells was used to generate cDNA (Superscript Choice System, Gibco BRL Life Technologies) with T7-(dT) 24 primers. Biotin-labelled ribonucleotides were synthesized using a BioArray high-yield RNA transcript labelling kit (Enzo Diagnostic Inc.) and hybridized onto the human Genome U133 Plus 2.0 chip (Affymetrix Inc.). Gene expression data network and enrichment analysis of the gene list was performed using MetaCore from GeneGo Inc. ( http://www.genego.com/metacore.php ). Human chemokine and cytokine antibody arrays Human cytokine antibody arrays (C Series 4000, Ray Biotech Inc.) were used according to the manufacturer’s instructions [65] . In brief, serum-free media from CAF cultures, CLS1/CAF co-cultures and CLS1 cultures were collected and incubated with the blocked membranes for 24 h at 4 °C with gentle shaking. After development, the chemiluminescent signals were captured using the Fujifilm LAS 3000 system (Fujifilm, Tokyo, Japan), and the images were processed with ImageJ software. The intensity of the chemiluminescent signal was normalized to that of the internal positive control. Western blot analyses The detailed procedures were performed as described previously [66] . The primary antibodies for p-IGF1R (Y1316, 6113S; 1:1,000), p-AKT (D9E; 1:1,000), AKT (927L; 1:1,000) and Nanog (D73G4; 1:1,000) were purchased from Cell Signaling Technology Inc., and the primary antibody for IGF1R (C-20; 1:1,000) was purchased from Santa Cruz. Monoclonal mouse anti-β-actin (Chemicon, Millipore; 1:5,000) was used as a loading control. The membranes were then washed three times with TBST, followed by incubation with horseradish peroxidase (HRP)-conjugated secondary antibody (1:5,000) in TBST/2% skim milk. Bound antibody was detected using the enhanced chemiluminescence system (Santa Cruz, CA). Chemiluminescent signals were captured using the Fujifilm LAS 3000 system (Fujifilm). All experiments were performed at least three times in duplicate. Full-length images of immunoblots are shown in Supplementary Fig. 16 . Patients and tumour specimens Lung tumour tissue specimens were obtained from patients ( N =80) with histologically confirmed NSCLC who had undergone complete surgical resections at the National Taiwan University Hospital (Taipei, Taiwan) between 28 December 1995 and 26 December 2005. This investigation was approved by the Institutional Review Board of the National Taiwan University Hospital (201103028RC). The enrolled patients were classified as stage I, and they had not been previously treated with neoadjuvant chemotherapy or irradiation therapy. All patients provided informed consent. All specimens were formalin fixed, sectioned, stained with haematoxylin and eosin and examined through microscopy. Pathological staging was performed by Dr Chang according to the international staging system for lung cancer [67] . IHC analysis tumour samples from lung cancer patients The detailed procedures were performed as described previously [68] and modified as the following procedures. IHC staining of tumour tissue samples from patients with NSCLC was performed using a modified UltraVision quanto HRP-diaminobenzidine detection system (Thermo, UK). The sections used for IHC analysis of IGF-II, IGF1R, Nanog and proliferating cell nuclear antigen (PCNA) protein expression were first autoclaved in Antigen Retrieval AR-10 Solution (BioGenex) or Antigen Retrieval Citra Solution (BioGenex) at 121 °C for 10 min. The samples were then treated with 3% H 2 O 2 -methanol and sequentially subjected to incubation with Ultra V Block (Lab Vision Corporation) for 10 min and incubation with a polyclonal anti-IGF-II antibody (MBS551011, MyBioSource; 1:100), a polyclonal anti-IGF1R-β antibody (#3027, Cell Signaling; 1:20), a rabbit monoclonal anti-Nanog (D73G4, Cell Signaling; 1:300) and mouse monoclonal anti-PCNA (PC-10, Thermo Scientific; 1:400) for 2 h at room temperature. Detection of the immunostaining was performed using the Super Sensitive Non-Biotin Polymer HRP Detection System (BioGenex), according to the manufacturer’s instructions. Statistical analysis The Kaplan–Meier method was used to estimate overall or relapse-free survival curves and the log-rank test was performed to test the difference between survival curves. Cutoff values for separations of high/low-risk groups were median of risk scores. The multivariable Cox proportional hazards regression analysis with covariates such as age, gender, cell type, tumour size, tumour grade, PCNA as a proliferative marker, IGF-II expression (high versus low), IGF1R expression (high versus low) and Nanog expression (high versus low) was used to evaluate the independent prognostic factors. The quantitative in vitro and in vivo data are presented as the mean±s.d. unless otherwise noted. Student’s t -tests were used in two-group comparison. One-way or two-way analysis of variance methods with Tukey’s post hoc correlations were used for multiple groups comparisons. All tests were two-tailed and P values <0.05 were considered significant. Accession codes: The microarray data for CAF, CLS1/CAF and CLS1 have been deposited in the NCBI Gene Expression Omnibus ( http://www.ncbi.nlm.nih.gov/geo/ ) under the accession code GSE38678 . How to cite this article: Chen, W.-J. et al. Cancer-associated fibroblasts regulate the plasticity of lung cancer stemness via paracrine signalling. Nat. Commun. 5:3472 doi: 10.1038/ncomms4472 (2014).